Robust spin crossover and memristance across a single molecule A nanoscale molecular switch can be used to store information in a single molecule. Although the switching process can be detected electrically in the form of a change in the molecule′s conductance, adding spin functionality to molecular switches is a key concept for realizing molecular spintronic devices. Here we show that iron-based spin-crossover molecules can be individually and reproducibly switched between a combined high-spin, high-conduction state and a low-spin, low-conduction state, provided the individual molecule is decoupled from a metallic substrate by a thin insulating layer. These results represent a step to achieving combined spin and conduction switching functionality on the level of individual molecules. Molecular electronics describes how the function of an electronic component is achieved using a single molecule [1] . For instance, molecular switches [2] may serve as high-density memory devices. As a promising molecular class, spin-crossover (SCO) complexes [3] contain a transition metal ion that can be switched between a low-spin (LS) and a high-spin (HS) state by external stimuli as temperature, light, pressure, magnetic or electric fields or charge flow [4] , [5] , [6] , [7] , [8] , [9] , [10] . The two configurations may lead to different conductances but, more importantly, the switchable spin of the metal ion has a high potential for molecular spintronics [11] . The SCO property is related to a delicate energy balance between the HS and LS state associated with conformational changes of the molecule. Maintaining this delicate balance for SCO molecules adsorbed onto surfaces requires carefully controlling the molecule′s interaction with the adjacent electrodes to sustain the SCO property. As a prototypical SCO complex [3] , Fe(1,10-phenanthroline) 2 (NCS) 2 molecules (Fe-phen) shown in Fig. 1a exhibits a LS→HS transition when heated above T C ≈175 K that is accompanied by a change in the Fe-N bond distances and angles [12] , leading to a reduction in the ligand fields around the Fe site. At low temperatures, the splitting Δ between the t 2g and the e g states is so large that Hund′s rules are broken and a LS state with S =0 is formed. At high temperatures, the ligand field is reduced and Hund′s rules yield a HS state with S =2 ( Fig. 1b ) [13] . Thermally induced switching may occur in bulk [3] or thick Fe-phen films [14] . Yet investigations on the SCO of individual molecules require a fixed temperature and single-molecule selectivity. In this sense, light-induced transitions are impractical because one cannot focus the stimulus by light on a single molecule within a dense molecular matrix. Using scanning tunnelling microscopy (STM), the stimulus can, however, be focused on the area of current flow, which is typically of nanometre size. Thus, with STM individual molecular switches can be addressed and reversibly switched, as well as the molecular origin of the switching event can be probed [2] . 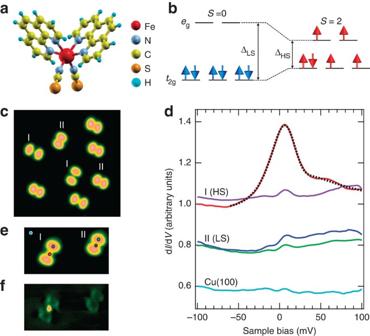Figure 1: SCO Fe-phen molecules on bare Cu(100). (a) Three-dimensional model of a Fe-phen molecule. (b) Simplified electronic configuration of the Fe(II) 3d states in the ligand field. For large ligand fields (ΔLS), the electrons fully occupy thet2gstates and the total spinSis quenched, while for low ligand fields (ΔHS), the Fe(II) ion is in the spin stateS=2. (c) STM image of isolated Fe-phen molecules on the Cu(100) surface with two conformations denoted as I (HS) and II (LS). Image size is 13×13 nm2. (d) dI/dVspectra recorded on the centre of type I (HS), type II (LS) molecules and Cu(100) surface. The colours indicate the position, where the spectra were taken and are marked as coloured dots of (e). The black dotted line denotes a Fano fit to the Kondo resonance. (e) STM topography of a pair of type I (HS) and type II (LS) molecules and (f) corresponding dI/dVmap (bottom) obtained at +10 mV showing the position of the Kondo resonance at the centre of the HS molecule. Image sizes are 6.7×3.7 nm2. Figure 1: SCO Fe-phen molecules on bare Cu(100). ( a ) Three-dimensional model of a Fe-phen molecule. ( b ) Simplified electronic configuration of the Fe(II) 3d states in the ligand field. For large ligand fields (Δ LS ), the electrons fully occupy the t 2 g states and the total spin S is quenched, while for low ligand fields (Δ HS ), the Fe(II) ion is in the spin state S =2. ( c ) STM image of isolated Fe-phen molecules on the Cu(100) surface with two conformations denoted as I (HS) and II (LS). Image size is 13×13 nm 2 . ( d ) d I /d V spectra recorded on the centre of type I (HS), type II (LS) molecules and Cu(100) surface. The colours indicate the position, where the spectra were taken and are marked as coloured dots of ( e ). The black dotted line denotes a Fano fit to the Kondo resonance. ( e ) STM topography of a pair of type I (HS) and type II (LS) molecules and ( f ) corresponding d I /d V map (bottom) obtained at +10 mV showing the position of the Kondo resonance at the centre of the HS molecule. Image sizes are 6.7×3.7 nm 2 . Full size image Here we demonstrate how to electrically switch the spin state of, and the conductance across, individual Fe-phen molecules using STM at low temperature (≈4.6 K) with high lateral and energy resolution. While Fe-phen molecules adsorbed onto a Cu(100) surface exhibit a coexistence of HS and LS states, the strong coupling of the NCS group to the substrate prevents a spin state from being written electrically. Introducing an interfacial CuN layer, however, allows switching between the HS and the LS state. The combined changes in conductance and spin state demonstrate how to confer memristive to spintronic properties realising multifunctional spintronic capacity in single molecules [11] , [15] . Fe-phen molecules on Cu(100) Figure 1c displays an STM image of isolated Fe-phen molecules on Cu(100). Each molecule shows two lobes. Because of the strong affinity of S to the Cu substrate, the NCS groups bind to the substrate and the two phen groups point upwards and are seen with the STM as the two lobes. There exist two molecular conformations for Fe-phen on Cu(100). Type I shows a larger inter-lobe distance than type II. To identify the spin state of the two types, differential conductance spectra of the tunnelling current (d I /d V ) were measured ( Fig. 1d ). The spectrum measured atop a type II molecule′s centre exhibits only minor differential conductance variations that are likely related to the electronic structure of the molecule adsorbed on Cu(100). In contrast, the spectrum atop a type I molecule′s centre shows a strong resonance near the Fermi energy. The resonance exhibits a Fano line shape [16] , indicating a Kondo resonance. A Fano fit to the spectrum reveals a Kondo temperature T K of ≈317 K, a q -factor of 6.1 and a shift of the Kondo resonance due to Coulomb repulsion of 5.7 meV. This large T K underscores a strong electronic hybridization between the Fe spin and the Cu substrate similar to that found in Fe 2+ ions of Fe-Phthalocyanine on Au(111) with Kondo temperatures between 357 and 598 K [17] . A d I /d V map of the Kondo feature ( Fig. 1e,f ) reveals that the Kondo cloud is centred around the expected position of the Fe-ion for a type I molecular conformation, while there is no resonance for a type II molecular conformation. A Kondo resonance is a signature of unpaired spins and is caused by a many-body state including the substrate electrons. Thus, these spectroscopic experiments ascribe a type I molecular conformation as the HS and type II as the LS state. As further evidence, we have carried out X-ray absorption spectroscopy (XAS) measurements of ≈2 molecular layers (ML) of Fe-phen on Cu(100) at low temperatures. As XAS is an element-specific spectroscopic method, this approach is very effective to elucidate the electronic structure of Fe ions, that is, to resolve the HS and LS states. During the measurements, no external illumination except for the X-rays was applied to avoid light-induced excited spin state trapping [18] . The surface structure of 2 ML thin films as verified by STM ( Supplementary Fig. S1a,b ) exhibits an ordered structure along the four-fold symmetry of the Cu(100) surface. A closer look at the film reveals the existence of two types of molecular conformations that are similar to the type I and type II conformations of individual molecules on Cu(100) shown in Fig. 1c . We first present XAS spectra of Fe-phen powder acquired above and below the SCO transition at T ≈175 K [14] , as references to analyse thin film data. Top and middle of Fig. 2a display the XAS spectra of the HS state and the LS state measured at 200 K and 100 K, respectively. Clear differences exist between the spectra, such as a dominant peak located at ≈706 eV for the HS state and at ≈708 eV for the LS state of the Fe 2p L 3 absorption edge, in good agreement with previous studies [19] . The bottom of Fig. 2a displays the XAS spectrum of the molecular film on Cu(100) measured at 50 K. In agreement with the STM experiments, the XAS spectrum exhibits both peaks indicating the coexistence of the two spin states. To confirm this interpretation, we have reproduced the XAS 2 ML spectrum through a linear combination of the HS (46% weight) and LS state (54% weight) reference spectra at the L 3 and the L 2 edge ( Fig. 2b,c ). The validity of the mixed spin state in 2 ML Fe-phen thin film is further reinforced by X-ray magnetic circular dichroism (XMCD) measurements showing nearly identical spectra for the thin film sample ( Fig. 2d ) and the powder sample ( Fig. 2e ). Note that some of the LS state molecules are switched to the HS state owing to the soft X-ray-induced excited spin state trapping [19] , which can be seen in the XAS spectra. A spectrum change of XAS with respect to circular right- and left- polarized X-ray was observed only near the peak at ≈706 eV and no change was observed at ≈708 eV. This clearly proves the coexistence of the two spin states, as the polarization of the X-ray only affects the magnetic HS state spectrum mainly positioned at ≈706 eV and the non-magnetic LS state spectrum mainly positioned at ≈708 eV does not react to the polarization of the X-ray. To conclude this part, XAS and XMCD measurements obtained on thin films on Cu(100) show that the spectra are split into two contributions very similar to those obtained for the HS and the LS states in bulk samples. Thus, the two molecular states observed in STM can be assigned to the HS ( S =2) and LS ( S =0) states. 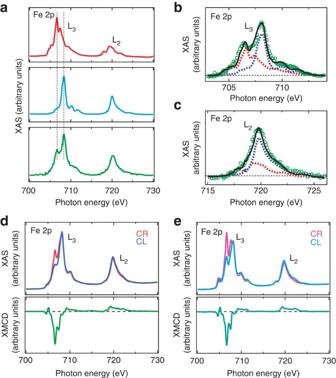Figure 2: Coexistence of HS and LS states of Fe-phen molecules on Cu(100). (a) Fe 2p XAS spectra of Fe-phen powder reference sample obtained at 200 K (HS state: top) and 100 K (LS state: middle), and two monolayers of Fe-phen thin film on Cu(100) obtained at 50 K (bottom). Reproduction of Fe 2p XAS L3(b) and L2(c) edges of two monolayers Fe-phen using the reference spectra for the HS and LS states obtained on the powder sample. Green circles represent the experimental data of the thin film, black lines the reproduced spectra obtained from the linear combination of the powder spectra of the HS state (red dotted line) and LS state (blue dotted line). The black dotted line represents the background. XAS and XMCD spectra of (d) two monolayers Fe-phen thin film on Cu(100) measured at 1.5 K and 6.5 T, and (e) Fe-phen powder reference sample measured at 4 K and 6.5 T. To obtain dichroic signal, the helicity of the X-ray was reversed between circular right (CR) and circular left (CL). The black dotted line shows the zero line of the XMCD signal. Figure 2: Coexistence of HS and LS states of Fe-phen molecules on Cu(100). ( a ) Fe 2p XAS spectra of Fe-phen powder reference sample obtained at 200 K (HS state: top) and 100 K (LS state: middle), and two monolayers of Fe-phen thin film on Cu(100) obtained at 50 K (bottom). Reproduction of Fe 2p XAS L 3 ( b ) and L 2 ( c ) edges of two monolayers Fe-phen using the reference spectra for the HS and LS states obtained on the powder sample. Green circles represent the experimental data of the thin film, black lines the reproduced spectra obtained from the linear combination of the powder spectra of the HS state (red dotted line) and LS state (blue dotted line). The black dotted line represents the background. XAS and XMCD spectra of ( d ) two monolayers Fe-phen thin film on Cu(100) measured at 1.5 K and 6.5 T, and ( e ) Fe-phen powder reference sample measured at 4 K and 6.5 T. To obtain dichroic signal, the helicity of the X-ray was reversed between circular right (CR) and circular left (CL). The black dotted line shows the zero line of the XMCD signal. Full size image Despite applying high local electric fields (up to several GV m −1 ) in the junction of the STM, high tunnelling voltages (± 4 V) and high current densities (up to 1 μA per molecule), we were unable to electrically switch between the two types ( Supplementary Fig. S2a–d ). Switching between the states was only possible by moving molecules laterally with the STM tip. We infer that the strong S-Cu bond impairs spin switching with the tunnelling conditions given above. Fe-phen molecules on CuN/Cu(100) To reduce the chemical interaction between molecule and substrate, we inserted a monoatomic CuN layer, which significantly reduces the adsorption energy and ensuing hybridization [20] . Moreover, the bond of S to the oxidized Cu atoms in the CuN network is expected to be weaker. 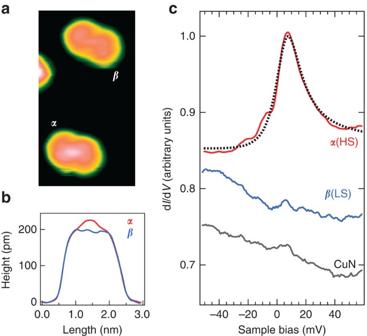Figure 3: SCO Fe-phen molecules on CuN/Cu(100). (a) STM image (3×5.5 nm2) of isolated Fe-phen molecules on the CuN/Cu(100) surface with two conformations denoted asα(HS) andβ(LS) and (b) line scans across the long axis of the molecules showing the difference in their appearance. (c) dI/dVspectra taken on the centre of the two configurations of the Fe-phen molecules together with a Fano fit (dotted black line) to the Kondo resonance of typeα. The black line is the spectrum recorded on bare CuN with the same tip. Figure 3a shows an STM image of isolated Fe-phen molecules on CuN/Cu(100). As with Cu(100), the STM images suggest that the molecules adsorb with the NCS groups onto the CuN surface, and two types of molecular conformations denoted as type α and type β are observed (for large-scale images of the CuN surface and the molecules on the CuN surface see Supplementary Fig. S3 a–d ). The difference in the molecular shape as seen by STM is significantly smaller when compared with that on bare Cu, which might be due to the electronic decoupling of the molecules. The two types reveal slight differences in the height profiles ( Fig. 3b ): the central region of type α is higher than that of type β . d I /d V spectra near the Fermi energy recorded on the centre of both types show a clear Kondo resonance only on type α and a weak spectroscopic feature on type β ( Fig. 3c ). A similarly weak feature is also frequently found in the spectrum recorded on bare CuN. We associate it with inelastic vibronic excitations of the CuN layer. From the spectroscopic data, we therefore ascribe the type α ( β ) as the HS (LS) conformational state in analogy to the molecules on Cu(100). As further confirmation, spectral data recorded on the organic ligands reveal strong electronic differences between the two types ( Supplementary Fig. S4 ), in agreement with theoretical predictions of electronic differences between the HS and LS molecules [12] . The weaker electronic hybridization expected on CuN compared with Cu results in a lowering of the fitted Kondo temperature to T K ≈105 K ( q =4.9, Coulomb shift 5.5 meV). This reduced hybridization also results in molecular orbitals that are energetically better defined ( Supplementary Fig. S4 ). Note, however, that the molecular states are still rather broad. From the observed widths of the molecular states, lifetimes of these excited states between 2 and 5 fs can be estimated. These short lifetimes indicate an efficient hybridization of the molecular states with the substrate and exclude the possibility that the observed peak of HS molecules at the Fermi level is caused by a charged state of the molecule. Figure 3: SCO Fe-phen molecules on CuN/Cu(100). ( a ) STM image (3×5.5 nm 2 ) of isolated Fe-phen molecules on the CuN/Cu(100) surface with two conformations denoted as α (HS) and β (LS) and ( b ) line scans across the long axis of the molecules showing the difference in their appearance. ( c ) d I /d V spectra taken on the centre of the two configurations of the Fe-phen molecules together with a Fano fit (dotted black line) to the Kondo resonance of type α . The black line is the spectrum recorded on bare CuN with the same tip. Full size image Contrary to Fe-phen on bare Cu(100), Fe-phen on CuN/Cu(100) can be electrically switched between the HS and LS states reproducibly, leading to a single-molecule device whose state can be deterministically selected. When performing cyclic I ( V ) curves atop the molecule′s centre with the STM feedback loop opened, conformational switching can be seen as an abrupt jump in the I ( V ) curve [2] . 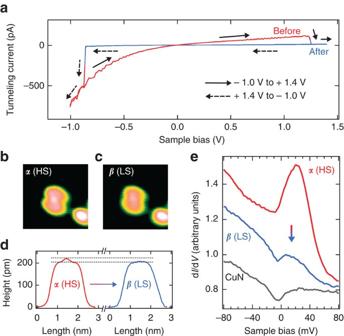Figure 4: Spin and junction conductance switching of single molecules. (a)I(V) curves of isolated Fe-phen molecules on the CuN/Cu(100) surface recorded on the centre of the molecule showing a hysteretic switching behaviour (tunnelling conditions for tip stabilization: +1 V, 100 pA). The high (red) and low (blue) junction conductance states are visualized using STM images (bfor HS state andcfor LS state, each 3.7×3.7 nm2) and corresponding height profiles (d) along the molecular long axis acquired before and after the switching event. (e) dI/dVspectra recorded on the centre of the molecule before and after a switching event from the high-conductance to the low-conductance state and spectrum of the bare CuN surface recorded with the same tip. (b) to (e) indicate that the switching event is a transition from the HS to the LS state. Figure 4a displays a typical cyclic I ( V ) sweep with arrows indicating the sweep direction. An abrupt current increase (decrease) is seen on the forward (reverse) sweep at ≈+1.2 V (≈−0.8 V). The cyclic I ( V ) curves depict a hysteretic behaviour at intermediate voltages indicated by two branches of the I ( V ) curve (high conduction branch in red and low conduction branch in blue). Repeated forward and reverse I ( V ) sweeps reveal the switching between the two states to be fully reversible. Figure 4: Spin and junction conductance switching of single molecules. ( a ) I ( V ) curves of isolated Fe-phen molecules on the CuN/Cu(100) surface recorded on the centre of the molecule showing a hysteretic switching behaviour (tunnelling conditions for tip stabilization: +1 V, 100 pA). The high (red) and low (blue) junction conductance states are visualized using STM images ( b for HS state and c for LS state, each 3.7×3.7 nm 2 ) and corresponding height profiles ( d ) along the molecular long axis acquired before and after the switching event. ( e ) d I /d V spectra recorded on the centre of the molecule before and after a switching event from the high-conductance to the low-conductance state and spectrum of the bare CuN surface recorded with the same tip. ( b ) to ( e ) indicate that the switching event is a transition from the HS to the LS state. Full size image This switching behaviour falls into the general category of memristive effects [21] , which generically describe how it is electrically possible to reversibly alter a device′s conductance. In our case, the two branches of the I ( V ) curve are related to the HS and LS states of the Fe-phen molecule as seen by comparing STM images and d I /d V spectra of the molecule in each of the two branches. When ramping the sample bias up, the molecule in the HS-state (type α ) is found to change its conformation after the abrupt drop in the tunnelling current to the LS-state (type β ), as shown in Fig. 4b and c with corresponding height profiles in Fig. 4d . This observation is reinforced by the associated changes in the d I /d V spectra ( Fig. 4e ). Equally, switching from the LS to the HS state has been verified. This unambiguously ascribes the intrinsic SCO property of Fe-phen as the origin of this nanoscale memristive behaviour. We exclude the possible artifact of STM tip changes, as the switching event does not alter the STM images and d I /d V spectra of the surrounding molecules. The observed combined switching of the spin and conduction state of the molecule is in line with recent predictions for similar molecules [22] . Note that SCO is not caused by charge transfer or unpaired spins on the organic ligands as in the case of switchable Kondo effect [23] , [24] . This is clearly evidenced by the fact that the Kondo resonance is only observed on the position of the central Fe ion and not on the organic ligands. Thus, the spin of the molecule is associated with a magnetic moment on the metal ion [3] . As the HS (LS) state of a single Fe-phen molecular junction can be prepared by applying a suitably large applied bias of negative (positive) polarity ( Fig. 4 ), we can test the bistable deterministic nature of this memory device by applying a suitable train of bias pulses. As shown in Fig. 5a , alternating positive and negative bias pulses lead to molecular junctions with a current level measured at +0.1 V that is associated with each of the desired LS and HS states, respectively. We emphasize that it is not only the amplitude of the bias pulse but also its polarity that determines the state after the pulse. After the molecule has been switched from the HS to the LS state by a positive voltage, it is not switched back by a second positive pulse to the HS state. Only applying a negative pulse switches the molecule back to the HS state ( Fig. 5b ). The same holds for the opposite switching process (not shown). This proves that addressing the memory device is fully deterministic. Furthermore, the lifetime of each spin state is remarkably long at the observation temperature: no spontaneous switches were observed even after tens of hours of STM observation at low bias voltages (<±0.5 V ). 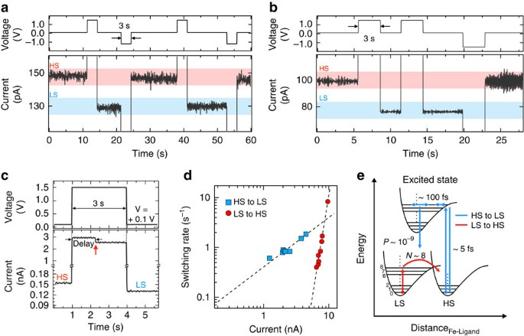Figure 5: Robust SCO-based single-molecule memristance. (a) Demonstration of reversible switching by voltage pulses of +1.5 V inducing HS to LS switching and −1.2 V inducing LS to HS switching. Corresponding to the polarity of the voltage pulse, the tunnelling current forV=+0.1 V is clearly switched between two levels corresponding to the HS and LS states (150 pA and 130 pA, respectively). The tip was initially stabilized at +100 mV and 150 pA. (b) Demonstration of deterministic switching by the application of two consecutive pulses of the same polarity. The first positive pulse switches the molecules from the HS to the LS state. The second positive pulse does not alter the state, while a third negative pulse switches back the molecule to the HS state. The tip was initially stabilized at +100 mV and 100 pA. (c) Real-time current trace of an isolated HS state molecule on the CuN/Cu(100) surface. A voltage pulse of +1.5 V is applied for 3 s and the transition to the LS state is witnessed by a small decrease in current after a delay of 1.4 s (red arrow). (d) Observed switching rates for HS to LS states and vice versa by voltage pulses of ±1.5 V. The dotted lines indicate power law fits of the switching as function of the absolute tunnelling current. (e) Proposed model for the switching mechanism in both directions. While the switching from the LS to the HS state is a high order process (N≈8) involving heating by the tunnelling electrons, the transition from the HS to the LS state only requires one electron (N≈1) and involves an intermediate short-lived excited state. Figure 5: Robust SCO-based single-molecule memristance. ( a ) Demonstration of reversible switching by voltage pulses of +1.5 V inducing HS to LS switching and −1.2 V inducing LS to HS switching. Corresponding to the polarity of the voltage pulse, the tunnelling current for V =+0.1 V is clearly switched between two levels corresponding to the HS and LS states (150 pA and 130 pA, respectively). The tip was initially stabilized at +100 mV and 150 pA. ( b ) Demonstration of deterministic switching by the application of two consecutive pulses of the same polarity. The first positive pulse switches the molecules from the HS to the LS state. The second positive pulse does not alter the state, while a third negative pulse switches back the molecule to the HS state. The tip was initially stabilized at +100 mV and 100 pA. ( c ) Real-time current trace of an isolated HS state molecule on the CuN/Cu(100) surface. A voltage pulse of +1.5 V is applied for 3 s and the transition to the LS state is witnessed by a small decrease in current after a delay of 1.4 s (red arrow). ( d ) Observed switching rates for HS to LS states and vice versa by voltage pulses of ±1.5 V. The dotted lines indicate power law fits of the switching as function of the absolute tunnelling current. ( e ) Proposed model for the switching mechanism in both directions. While the switching from the LS to the HS state is a high order process ( N ≈8) involving heating by the tunnelling electrons, the transition from the HS to the LS state only requires one electron ( N ≈1) and involves an intermediate short-lived excited state. Full size image To gain further insight into the switching mechanism, we have examined the real-time traces of the tunnelling current during the bias pulse used to perform switching (feedback loop opened). Within the bias pulse, the current from a typical trace exhibits a small stepwise reduction that occurs in the typical example shown in Fig. 5c after a time delay of 1.4 s. Thus, the switch does not occur instantaneously but after a significant delay. By performing many switching events, we have extracted the average switching rate as a function of the current during the pulse. As the linear fits (dotted lines) of the HS→LS and LS→HS switching rates versus current in Fig. 5d with logarithmic x - y scales show, a simple power law relates the rate R to the current I as R I N . We find that N ≈8 for the LS→HS transition, suggesting a higher-order process involving vibrational heating due to inelastic scattering of the tunnelling electrons [2] , [25] , in competition with a heat loss to the substrate. For the HS→LS transition, we find that the switching rate scales linearly with current ( N ≈1). This indicates that, although the switching probability per electron is on the order of P ~10 −9 , the switching is caused by single electron processes. We note that the HS→LS conformational switch at voltages above ≈+1.1 V could involve injecting charge onto the state that is present at +1.1 eV ( Supplementary Fig. S4 ). In the following, we discuss the broad features of a model for electrical molecular switching in analogy to that of optical switching. When exciting the molecule from the HS state with electrons to the molecular state at +1.1 V, the positions of the atomic cores are initially not changed owing to their slow reaction. This excited state can favour ligand's distances to the central Fe ion that better match those of the LS state. If the lifetime of the excited state were long, the excited state would relax into its vibronic ground state. Electronic deexcitation would then result in the LS state of the molecule ( Fig. 5e ). The spectroscopic data, however, indicate that the electronically excited state has a lifetime of only 5 fs. Yet typical vibration times of the vibronic excitations are in the range of 10 THz, that is, periods of a tenth of a ps. Thus, only in the low-probability case that the electronically excited state survives for 0.1 ps is a transition possible. A simple calculation for 5 fs electronic lifetime and 10 THz vibration frequency results in a switching probability of P =2×10 −9 . This naturally explains the low success rate for switching and agrees with the observed order of the process of N =1. Interestingly, the energy of the excited state in STM experiments lies close to that needed for optical switching (1.49 eV), which is associated to the transition of the molecule from the 5 T 2 to the 5 E state [4] . In this sense, a thicker insulating layer could increase the lifetime of the excited state and thus the switching probability. Further experiments, such as time-resolved optical pump probe measurements, could clarify the switching mechanism. In conclusion, once the molecule–electrode interaction is reduced, individual Fe-phen SCO molecules can be reversibly and deterministically switched by a STM to a specific spin state, leading to a large difference in junction conductance. More broadly, strategies within the past decade to combine memristive [21] , [26] and spintronic [15] functionalities in devices have relied on extrinsic [27] , [28] or nominally intrinsic [29] properties of the materials and interfaces within the device. Similar yet separated memristive [2] and spintronic [11] functionalities have arisen in the ultimate limit of single-molecule junctions. Our results show how to harness an unambiguously intrinsic property—SCO—to obtain memristive functionality. This functionality is robust, as it shows deterministic and reproducible switching depending on the polarity of the applied current, shows hysteresis and no spontaneous switches were observed for low tunnelling voltages. Relative to the SCO energy barrier, by appropriately tuning the hybridization strength of a SCO molecule adsorbed onto a suitable spin injector, one could also achieve spintronic functionality on a similar, single-molecule, magnetomemristive-based device potentially in spatially dense, multifunctional memory applications. During the refereeing of this manuscript, we became aware of a closely related work, which has been published in the meantime [30] . STM experiments STM measurements were carried out in a home-built STM [31] in ultra high vacuum ( p <2.0×10 −10 mbar) at low temperature (4.6 K). The STM tips were prepared by chemical etching of a tungsten wire and flashing in ultra-high vacuum. The clean and flat Cu(100) surface was prepared by several cycles of Ar + sputtering (1.5 keV) and subsequent annealing up to 450 °C. Fe(phen) 2 (NCS) 2 molecules were sublimed at 180 °C in ultra-high vacuum, while maintaining the Cu(100) and CuN/Cu(100) surfaces at room temperature. The differential conductance d I /d V spectra were obtained with a lock-in technique using a modulation bias of 3 mV and a frequency of 723 Hz. When ramping the voltage, the feedback loop was opened. X-ray absorption experiments Soft XAS and XMCD measurements were performed at the DEIMOS beamline of SOLEIL in France in total electron-yield mode at several temperatures and magnetic fields. The measurement chamber is connected to chambers allowing in situ preparation and characterization (Auger electron spectroscopy, STM) of the samples. Preparation of CuN layers To reduce the interaction between Fe-phen molecules and the substrate, one monolayer decoupling CuN film was introduced on Cu(100) surface. After obtaining a clean Cu(100) surface, the CuN layer was prepared by ionic bombardment at room temperature for 25 min. using 4×10 −4 mbar of N 2 , a beam energy of 500 eV and subsequent annealing up to 330 °C. With these preparation parameters, the entire Cu(100) surface is found to be covered with a CuN layer. How to cite this article: Miyamachi, T. et al . Robust spin crossover and memristance across a single molecule. Nat. Commun. 3:938 doi: 10.1038/ncomms1940 (2012).